Reversible control of magnetic interactions by electric field in a single-phase material Intrinsic magnetoelectric coupling describes the interaction between magnetic and electric polarization through an inherent microscopic mechanism in a single-phase material. This phenomenon has the potential to control the magnetic state of a material with an electric field, an enticing prospect for device engineering. Here, we demonstrate ‘giant’ magnetoelectric cross-field control in a tetravalent titanate film. In bulk form, EuTiO 3 , is antiferromagnetic. However, both anti and ferromagnetic interactions coexist between different nearest europium neighbours. In thin epitaxial films, strain was used to alter the relative strength of the magnetic exchange constants. We not only show that moderate biaxial compression precipitates local magnetic competition, but also demonstrate that the application of an electric field at this strain condition switches the magnetic ground state. Using first-principles density functional theory, we resolve the underlying microscopic mechanism resulting in G-type magnetic order and illustrate how it is responsible for the ‘giant’ magnetoelectric effect. The magnetoelectric (ME) effect represents the coupling between the electric and magnetic parameters in matter [1] . Multiferroic (MF) materials with coexisting ferromagnetism (FM) and ferroelectricity were thought to offer the best prospect of achieving a strong linear ME coupling coefficient owing to the combination of typically higher electric permittivity and magnetic permeability, both of which combine as an upper limit to any potential coupling strength [2] . Unfortunately, ME–MF materials are rare as ferroelectric materials need to be robustly insulating while magnetic materials are typically conducting [3] . Although uncommon, such compounds have been the subject of intense research over the past decade [1] , [2] . The realization of this phenomenon may lead to the development of multistate logic, new memory or advanced sensor technologies [2] . To integrate such characteristics into a functional device requires strong ME coupling between the ferroic properties, enabling the manipulation of magnetic order with an electric ( E ) field or electric polarity with a magnetic field. The intense search for materials exhibiting such functional ferroic control has centred upon a number of complex oxide systems with a pseudo-cubic perovskite structure [2] , [3] , [4] , [5] . Within these systems, the electronic band structure of the central B-site cation generally determines the ferroic properties. A completely empty d band is required for ferroelectricity, while partial occupation is essential for the double and superexchange (SE) magnetic interactions, typical of these materials [3] , [6] . One approach circumventing this obstacle has been to engineer spatially segregated two-phase systems, which take advantage of electro- or magneto-striction mediated through strain or proximity to generate ME coupling [7] , [8] , [9] , [10] , [11] , [12] . However, finding an intrinsic single-phase mechanism would evade the inherent disadvantages and complexities of multiphase environments. In single-phase systems, the d band occupation issue is typically avoided through geometric (magnetic) frustration, where the ferroic properties arise from the Dzyaloshinski–Moriya interaction [13] , [14] , [15] . In these cases, the ferroic properties are weak, relegating device application unlikely. Suffice to say, a great deal has been accomplished regarding E -field-controlled magnetism. The popular MF pseudo-perovskite material BiFeO 3 , which presents both G-AFM and ferroelectric order, has shown intrinsic single-phase ME character. The orientation of the AFM Fe spins are always perpendicular to its rhombohedral long axis, which derives from the ferroelectric distortion. As a result, the magnetic domain structure can be reoriented by E -field application [16] . Equally important, the manganite family has had a significant role in our understanding of ME phenomena. Interest peaked with HoMnO 3 , when FM, correlated with Ho 3+ spin ordering, was activated by a static E -field [17] . Interestingly, the induced FM order originated from uncompensated magnetization at the AFM domain walls rather than from an intrinsic phenomenon [18] , [19] . Similarly, cross-coupling effects were found in another single-crystal ferrite system, GdFeO 3 , arising from domain wall interactions when weak MF–FM domains interfaced with ferroelectric regions [12] . Designing epitaxial heterostructures have also generated several avenues creating coupled control parameters. Interfacing MF materials BiFeO 3 or YMnO 3 with a soft FM system provides opportunities for phase coupling to electrically control both magnetic exchange bias and spin reorientation [8] , [10] , [20] , [21] . In addition, more direct methods have included altering the ferroelectric domain orientation of a BaTiO 3 single crystal demonstrating the ability to change the magnetic strength of a FM La 0.66 Sr 0.33 MO 3 film [7] , and active strain tuning through interfacing the same material to a piezoelectric single crystal presented the ability to change the magnetic transition temperature, T C , with E -field [22] . The rare earth tetravalent titanate, EuTiO 3 (ETO), is an emerging multication ferroic prototype, whereby magnetic spins are carried by the half-occupied Eu 4f 7 spins, and the unoccupied Ti 3d 0 band lends itself to potential ferroelectricity. Moreover, the anomalous response of the dielectric constant to spin alignment indicates an inherent ME coupling mechanism in ETO ( [23] ). It was this effect that impelled Fennie and Rabe to calculate that, through strain engineering, one could create strong multiferroicity and additionally predicted the exceptional strain-boundary state, allowing cross-field control capability [24] . Indeed, epitaxial films of tensile-strained ETO showed multiferroicity with a large ferromagnetic moment (7 μ B /Eu) alongside spontaneous electric polarization (~10 μCm −2 ) ( [25] ). Furthermore, ETO demonstrates a third-order biquadratic ME coupling response ( E 2 H 2 ) allowing for circumvention of the linear ME susceptibility boundary condition [26] . In this article, we present E -field control of the full magnetic moment in the single-phase ETO system. However, our findings do not match initial predictions. Instead, we find that the dramatic ME effect does not require the proposed polar instability [24] . Rather, the combination of tuning the relative strengths of the intrinsic competing magnetic interactions under a moderate compressive strain state with the inherent paraelectric nature of the system is sufficient to generate complete ME control. X-ray resonant magnetic scattering (XRMS) was used to confirm the magnetic structure of the contrasting strained ETO film series and reveal the emergence of competition between coexisting magnetic interactions in a moderately (−0.9%) compressed state. First-principles density functional theory (DFT) calculations identified the third nearest neighbour (NN) Eu interaction central to the G-AFM structure of ETO. Finally, using in situ ( E -field) XRMS, we demonstrate cross-field ME control by eliminating long-range AFM order and inducing a magnetic state of nanometre-sized FM clusters. The underlying intrinsic mechanism is illustrated through simulations replicating the effect of E -field application by calculating the energy difference between the AFM and FM spin configurations. X-ray resonant magnetic scattering X-ray scattering is sensitive to both charge and magnetic distributions [27] . Typically, the magnetic component is about six orders of magnitude lower than conventional charge scattering. However, an enhanced magnetic response is achieved through resonance, in the present case at the Eu L II edge, whereby, mediated by the Eu 4f-5d exchange interaction, the Eu sublattice magnetic structure is probed with E1 (2p 1/2 –>5d 3/2 ) electronic excitations. In addition, owing to the polarization dependence of magnetic scattering a post-sample analyser can be used to preferentially suppress charge scattering as illustrated in Fig. 1a . Unstrained, compressive and tensile strain states were accomplished with 22 nm of epitaxial cube on cube-layered growth by ozone-assisted molecular beam epitaxy on SrTiO 3 (STO), (LaAlO 3 ) 0.29 −(SrAl ½ Ta ½ O 3 ) 0.71 (LSAT) and DyScO 3 (DSO) single-crystal substrates, respectively [25] . 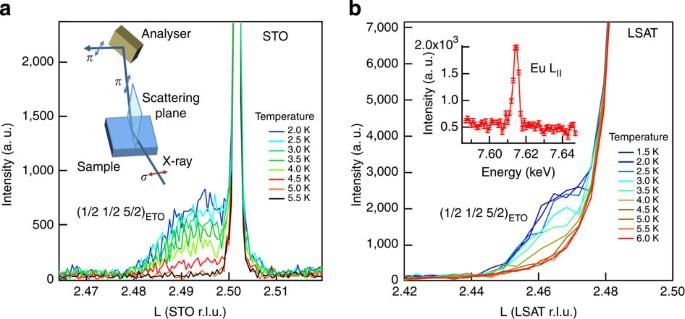Figure 1: XRMS spectra showing G-AFM order in epitaxial ETO films grown on STO(001) and LSAT (001) substrates. (a) A series of reciprocal L-scans (film normal) through the (1/2 1/2 5/2)ETOreflection of the nominally unstrained ETO on STO(001) through a range of temperatures crossingTN. Also seen is a half-order reflection from the STO substrate owing to AFD order. The measurements were taken in vertical scattering geometry with σ- to π-polarization selection analysis (inset) used to suppress charge and optimize the magnetic/charge scattering ratio. (b) A similar temperature-dependence data set for the compressively (−0.9%) strained ETO on LSAT(001). The encumbering substrate charge intensity originates from anti-phase boundary half-order reflections typical of LSAT. The inset shows the resonant response with an energy scan at 1.5 K through the Eu LIIedge. The error bars present s.d. Figure 1: XRMS spectra showing G-AFM order in epitaxial ETO films grown on STO(001) and LSAT (001) substrates. ( a ) A series of reciprocal L-scans (film normal) through the (1/2 1/2 5/2) ETO reflection of the nominally unstrained ETO on STO(001) through a range of temperatures crossing T N . Also seen is a half-order reflection from the STO substrate owing to AFD order. The measurements were taken in vertical scattering geometry with σ- to π-polarization selection analysis (inset) used to suppress charge and optimize the magnetic/charge scattering ratio. ( b ) A similar temperature-dependence data set for the compressively (−0.9%) strained ETO on LSAT(001). The encumbering substrate charge intensity originates from anti-phase boundary half-order reflections typical of LSAT. The inset shows the resonant response with an energy scan at 1.5 K through the Eu L II edge. The error bars present s.d. Full size image Both ETO and STO share the same lattice parameter, thus when grown on the (001) surface, the film is nominally unstrained and exhibits bulk like G-AFM order with the emergence of magnetic scattering intensity at (1/2 1/2 5/2) ETO below T N at 5.25 K shown in Fig. 1a . A −0.9% compressive strain is imposed by the LSAT (001) substrate and as shown in Fig. 1b also maintains G-AFM order with the onset of magnetic scattering at T N of 4.96 K. Under 1.1% tensile strain the ETO film grown on DSO(110) is, however, ferromagnetic, confirmed both by the absence of a resonant magnetic signature at the (1/2 1/2 5/2) ETO reflection shown in Fig. 2a and with the emergence of a resonant enhancement of the magnetic scattering at the (001) ETO reflection at the Eu L II edge shown in Fig. 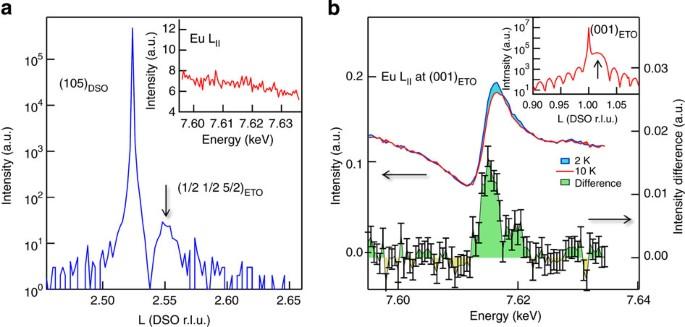Figure 2: XRMS showing absence of G-AFM order and emergence of FM order in 1.1% tensile-strained ETO on DSO(110) substrate. (a) An L-scan through the (1/2 1/2 5/2)ETOreflection at 1.6 K below theTCmark of 4.05 K. Some charge-scattered leakage is detected; however, an energy scan through the Eu LIIedge is presented in the inset showing no resonant (magnetic) response. The finding demonstrates absence of long-range G-AFM order of the Eu ions in the FM phase. The leaked charge amplitude derives from the octahedral tilting pattern, (a−a−c0) (ref.32). (b) Presents contrasting energy scans through the Eu LIIedge above and belowTCat the integer (001)ETOreflection. Inset plots an L-scan through the same reflection. Owing to the overlap of both charge and magnetic scattering at this reflection, complete suppression of the former is constrained. The onset of magnetic scattering belowTCis shown with the increase of scattered intensity through the edge and indicates the spontaneous (zero field) FM long-range order. The magnetic scattering contribution was about 9% of the total intensity. The results of statistical error propagation is presented for the difference signal. 2b , with a T C of 4.05 K. Figure 2: XRMS showing absence of G-AFM order and emergence of FM order in 1.1% tensile-strained ETO on DSO(110) substrate. ( a ) An L-scan through the (1/2 1/2 5/2) ETO reflection at 1.6 K below the T C mark of 4.05 K. Some charge-scattered leakage is detected; however, an energy scan through the Eu L II edge is presented in the inset showing no resonant (magnetic) response. The finding demonstrates absence of long-range G-AFM order of the Eu ions in the FM phase. The leaked charge amplitude derives from the octahedral tilting pattern, (a − a − c 0 ) (ref. 32 ). ( b ) Presents contrasting energy scans through the Eu L II edge above and below T C at the integer (001) ETO reflection. Inset plots an L-scan through the same reflection. Owing to the overlap of both charge and magnetic scattering at this reflection, complete suppression of the former is constrained. The onset of magnetic scattering below T C is shown with the increase of scattered intensity through the edge and indicates the spontaneous (zero field) FM long-range order. The magnetic scattering contribution was about 9% of the total intensity. The results of statistical error propagation is presented for the difference signal. Full size image Contrasting with the unstrained (STO) and tensile strain (DSO) conditions, the temperature dependence of the magnetic scattering intensity of the compressive state (LSAT) shows a significantly dissimilar and suppressed critical behaviour, presented in Fig. 3a . This character is found in systems owing to local competition between FM and AFM interactions exemplified by the mixed-magnetic crystal system Gd x Eu 1−x S ( [28] ). The temperature-dependent magnetic scattering intensity is fit to the critical behaviour ‹ m › 2 ~ I = I 0 (1− T / T C ) 2 β , where ‹ m › is the magnetic moment, I is the magnetic scattered intensity, T is the sample temperature, T C is the magnetic transition temperature and β is the the critical order exponent. The AFM order of the ETO on STO film is best described by the three-dimensional Heisenberg model owing to the isotropic (rotational degree of freedom) character of half-filled Eu 4f spin states. The measured critical order exponent, β =0.385 of the same film follows ‘universally’ within the framework of statistical mechanics. However, a larger exponent, 0.496, is found in the compressively strained ETO film on LSAT (001). The substantial magnetic suppression demonstrates significant local magnetic competition. Similar to the unstrained G-AFM state, the tensile-strained ETO–DSO film in the FM phase also indicates three-dimensional Heisenberg behaviour where the local FM exchange dominates the AFM interactions without evidence of competing magnetic interactions. 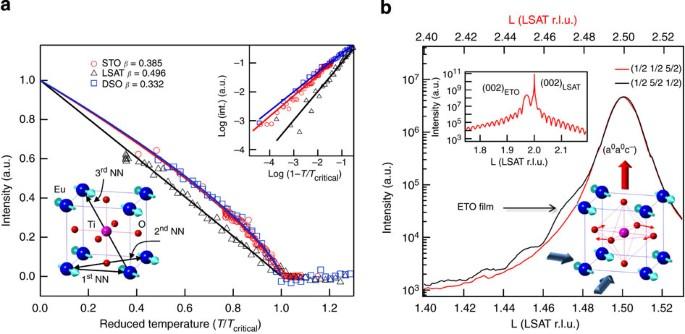Figure 3: Magnetic critical behaviour of the three strain states and XRD of the oxygen octahedral rotations in the ETO on LSAT. (a) The temperature dependence of the XRMS Eu LIIamplitudes for all three strain states, STO—unstrained, LSAT—0.9% compressive and DSO—1.1% tensile. The solid lines are fits of the critical behaviour ‹m›2~I=I0(1−T/TC)2β, where ‹m› is the magnetic moment,Iis the magnetic scattered intensity,Tis the sample temperature,TCis the magnetic transition temperature andβis the critical order exponent. Both the G-AFM order in the unstrained (STO) and FM order of tensile (DSO) films show typical three-dimensional Heisenberg behaviour while the compressively strained (LSAT) film shows significant suppression, a classic indicator of local magnetic competition. Inset—top, presents a log–log plot showing the near transition region. Inset bottom illustrates the multiple coexisting magnetic interactions between the first, second and third NN Eu ions. (b) The symmetry response of the ETO film to the biaxial compressive tetragonal distortion imposed by the LSAT (001) substrate. Both the (1/2 5/2 1/2)ETOand (1/2 1/2 5/2)ETOreflections at 300 K are presented. The occurrence of half-order Bragg peaks show the presence of long-range AFD rotations in the film. The combination of H=L allowed and H=K forbidden reflections indicate I4/mcm symmetry with the oxygen octahedral pattern (a0a0c−) in Glazer notation32, illustrated in the bottom inset. Again the LSAT substrate generates substantial background from the anti-phase boundary half-order reflections. The top inset indicates the relative position of the (002)ETOreciprocal position with respect to the substrate (002)LSAT. Figure 3: Magnetic critical behaviour of the three strain states and XRD of the oxygen octahedral rotations in the ETO on LSAT. ( a ) The temperature dependence of the XRMS Eu L II amplitudes for all three strain states, STO—unstrained, LSAT—0.9% compressive and DSO—1.1% tensile. The solid lines are fits of the critical behaviour ‹ m › 2 ~ I = I 0 (1− T / T C ) 2 β , where ‹ m › is the magnetic moment, I is the magnetic scattered intensity, T is the sample temperature, T C is the magnetic transition temperature and β is the critical order exponent. Both the G-AFM order in the unstrained (STO) and FM order of tensile (DSO) films show typical three-dimensional Heisenberg behaviour while the compressively strained (LSAT) film shows significant suppression, a classic indicator of local magnetic competition. Inset—top, presents a log–log plot showing the near transition region. Inset bottom illustrates the multiple coexisting magnetic interactions between the first, second and third NN Eu ions. ( b ) The symmetry response of the ETO film to the biaxial compressive tetragonal distortion imposed by the LSAT (001) substrate. Both the (1/2 5/2 1/2) ETO and (1/2 1/2 5/2) ETO reflections at 300 K are presented. The occurrence of half-order Bragg peaks show the presence of long-range AFD rotations in the film. The combination of H=L allowed and H=K forbidden reflections indicate I4/mcm symmetry with the oxygen octahedral pattern (a 0 a 0 c − ) in Glazer notation [32] , illustrated in the bottom inset. Again the LSAT substrate generates substantial background from the anti-phase boundary half-order reflections. The top inset indicates the relative position of the (002) ETO reciprocal position with respect to the substrate (002) LSAT . Full size image DFT calculations Clearly both local AFM and FM interactions coexist within the ETO. In order to describe the underlying mechanism determining the G-AFM Eu spin structure, previous first-principles DFT focused on the first and second NN Eu ion interactions, illustrated in Fig. 3a —inset [29] , [30] . Without significant volume (lattice) expansion, the calculations found FM order preferential. However, to investigate the underlying factor leading to the G-AFM magnetic structure, the issue of symmetry needed to be addressed, in order to best know the structure at hand. This was accomplished through a combination of DFT calculations and X-ray diffraction (XRD) measurements. Until recently, bulk EuTiO 3 under zero stress boundary conditions was traditionally believed to be in high-symmetry cubic Pm-3m space group. However, our first-principles calculations indicated that there were strong rotational instabilities as recently discussed by Rushchanskii et al . [31] With full ionic relaxation, we show that the lowest energy structure is I4/mcm or (a 0 a 0 c − ) in Glazer notation with the emergence of antiferrodistortive (AFD) oxygen octahedral rotations [32] . The energy gained from this distortion is 30 meV f.u. −1 (formula unit); however, the energy difference between this state and another metastable state, Imma, (a − a − c 0 ), is less than an meV f.u. −1 The competition between these two possible rotation patterns becomes evident when we consider the structures under strain. To simulate strain, geometric relaxations were performed keeping the in-plane lattice constant fixed and relaxing the out-of-plane lattice length corresponding to the films fixed biaxial boundary conditions. When we compare energies of different rotation patterns under these conditions, the two aforementioned patterns compete. Consequently the (a − a − c 0 ) pattern is favoured under tensile strain and (a 0 a 0 c − ) is preferred under compressive strain. XRD confirmed the I4/mcm symmetry in the compressed ETO film on LSAT(001).The combination of the non-zero H = L (1/2 5/2 1/2) ETO reflection with the absence of the H = K (1/2 1/2 5/2) ETO peak presented in Fig. 3b indicates the emergence of a pure in-plane AFD rotation finding agreement with the DFT calculations [33] . Including the octahedral rotations in our DFT calculations increases the compressive strain required to induce the predicted polar instability [24] . The competitive coupling between the polar and rotational structural instabilities leads to the calculated suppression of the phonon instability state [34] . The biaxial compression drives the AFD in-plane rotation in an attempt to maintain the Ti–O bond lengths, consequently preventing the T01 phonon from ‘freezing’ out of the film plane by providing a mechanism to minimize bond length changes. While the previous calculations without rotations (pm-3m) indicated a ~−0.9% strain generating the polar instability, our current calculations, including the AFD rotations, require ~−2.5% compressive strain beyond what is currently achievable. In Table 1 , we present the calculated results of the magnetic exchange interactions ( J ) for the first, second and third NN Eu ions for the ETO I4/mcm structure for both bulk (zero boundary conditions) and under −0.9% compressive strain, simulating epitaxial growth on the LSAT substrate. The exchange constants are broken down further into in-plane ( xy ) and out-of-plane ( z ), with positive and negative values indicating FM and AFM, respectively. We find that both the first and second NN Eu atoms interact in aggregate, with FM order. The third NN interaction, however, is AFM coupled. This diagonal exchange is most likely facilitated by the central Ti 3d 0 band coupled to the Eu 4f 7 spins through a 180° SE mechanism mediated by the intra-atomic-hybridized 4f-5d orbitals, similar to the previously proposed 90° SE mechanism between the first NN Eu ions [29] . As a result, the G-AFM structure is dependent upon this third NN interaction. Moreover, the strength of this SE coupling is reliant upon the Eu–Ti–Eu bond alignment and the degree of interatomic orbital overlap, thus sufficient angular distortion could significantly alter the magnetic structure of the entire system [35] . Table 1 Calculated magnetic exchange constants. Full size table Applying electric fields Upon this premise, the paraelectric nature of the ETO film becomes central to the feasibility of ME control. In Fig. 4a , the cartoon illustrates how the third NN interaction bond angle alignment is distorted by the Ti displacement from its central position under an applied E -field, reducing the efficacy of the interaction. Under biaxial compression, the system is expected to have a preferential uniaxial polar anisotropy with the Ti displacement out of the film plane. Thus in order to examine the capability of ME cross-field control, we measured the magnetic signature of the strained ETO–LSAT film where the competition between the magnetic interactions is prevalent and applied an E -field across the film to further alter the magnetic balance, as illustrated in the sample schematic in Fig. 4b . 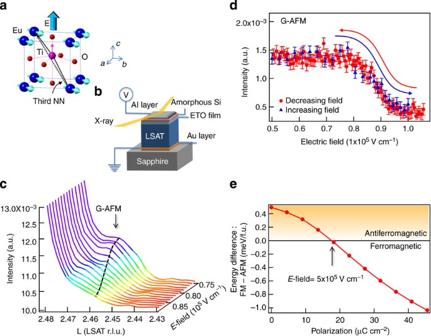Figure 4: Electric field control of the magnetic state. (a) The response of the Ti atom toE-field is represented pictorially as a displacement along the direction of the field distorting the Eu–Ti–Eu third NN bond alignment. (b) Presents a schematic of the experimental sample environment for thein situXRMS measurement. The sample is mounted on a sapphire block to achieve electrical isolation and maintain good thermal conductivity. (c) A series of L-scans through the G-AFM scattered (1/2 1/2 5/2)ETOreflection with incrementally increasingE-field strength showing the suppressive response of the AFM signature. (d) Presents a staticQplot of the magnetic scattering intensity (1/2 1/2 5/2)ETOversusE-field with increasing and decreasing field strength. The error bars represent the s.d. (e) A plot of the first-principles DFT calculations of the energy differences between FM and G-AFM spin configurations as a function of polarization modelled upon the ETO on LSAT with a compressive strain state of −0.9% and (a0a0c−) octahedral symmetry34. The calculation replicates the suppression of the AFM state in agreement with the experimental observation. Figure 4: Electric field control of the magnetic state. ( a ) The response of the Ti atom to E -field is represented pictorially as a displacement along the direction of the field distorting the Eu–Ti–Eu third NN bond alignment. ( b ) Presents a schematic of the experimental sample environment for the in situ XRMS measurement. The sample is mounted on a sapphire block to achieve electrical isolation and maintain good thermal conductivity. ( c ) A series of L-scans through the G-AFM scattered (1/2 1/2 5/2) ETO reflection with incrementally increasing E -field strength showing the suppressive response of the AFM signature. ( d ) Presents a static Q plot of the magnetic scattering intensity (1/2 1/2 5/2) ETO versus E -field with increasing and decreasing field strength. The error bars represent the s.d. ( e ) A plot of the first-principles DFT calculations of the energy differences between FM and G-AFM spin configurations as a function of polarization modelled upon the ETO on LSAT with a compressive strain state of −0.9% and (a 0 a 0 c − ) octahedral symmetry [34] . The calculation replicates the suppression of the AFM state in agreement with the experimental observation. Full size image A series of reciprocal space scans through the G-AFM (1/2 1/2 5/2) ETO magnetic reflection at 1.9 K versus E -field strength is presented in Fig. 4c . The suppression of the XRMS intensity with E -field is clearly displayed and is ostensibly eliminated by 1.0 × 10 5 V cm −1 . The transition lacks hysteresis, is continuous and reproducible. In Fig. 4d , the resonant magnetic scattering amplitude at the fixed film Q position is plotted with decreasing E -field strength and on the return the data are extracted from a series of L scans through the magnetic reflection at each field point. This plot exemplifies the reversibility and demonstrates the stability of the transition with each data point separated by 30 min on the return. To further establish the proposed underlying ME microscopic mechanism, we performed first-principles DFT calculations to replicate the response of the applied E -field on the strained film. In Fig. 4d , the calculated enthalpy difference between the G-AFM and FM spin configurations is plotted against the effective polarization. The simulation calculates the lowest-frequency polar Eigen mode, and forcibly displaces the oxygen ions incrementally further from the face centre in conjunction with the Ti shift to maintain this frequency minimum. The resulting energy differences between both magnetic states are calculated. The system responds by energetically trending from AFM towards FM order with increasing polarization. Crucially, it is the paraelectric ground state that allows for the ability to displace the Ti atom. This shift affects the relative strength of the local magnetic interactions reducing the third NN exchange coupling. This phenomenon is underpinned by the spatial overlap between the Eu 5d and Ti 3d orbitals, and their energetic degeneracy that is intricately balanced so that a small ionic displacement has a significant effect on the AFM strength. In order to reach a quantitative correlation between experiment and theory, we have estimated the critical E -field by dividing the energy required to displace the ions by the polarization. To generate a polarization field of P =18 μC cm −2 , where AFM and FM states are degenerate, would require ~5 × 10 5 V cm −1 . This is comparable to the experimental field found to extinguish the AFM state, ~1.0 × 10 5 V cm −1 . X-ray resonant interference scattering To explore the ensuing magnetic state by E -field, we employed X-ray resonant interference scattering (XRIS) [36] . XRIS is sensitive to the magnetic moment aligned along one direction by either an internal FM interaction or an external magnetic field. Even in the AFM state, the magnetic moments uniformly canting towards an external magnetic field direction result in charge–magnetic interference of the scattered intensity illustrated in Fig. 5a . Here, contrasting energy scans through the Eu L II edge at the (003) ETO reflection with opposing applied magnetic field directions ([110] ETO ) at 1.2 T in the film plane demonstrate the interference effect. The measurements were made in horizontal scattering geometry, which provides for additional charge scattering suppression, illustrated in Fig. 5b –inset. In ETO, the AFM coupling is generally weak and as a result 1 T is sufficient to fully saturate the Eu moments along the magnetic field direction shown by the magnetic field dependence of the interference effect in Fig. 5b . This plot shows that the degree of magnetic moment canting by the external H -field is proportional to the field strength. 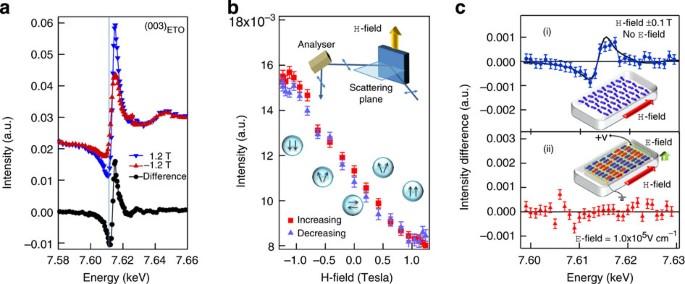Figure 5: The response of Eu spin alignment with appliedH-field in the ETO film on LSAT with and withoutE-field. (a) Energy scans through the Eu LIIedge at the (003)ETOreflection with ±1.2 T showing the maximum interference effect at full saturation between the magnetic and charge scattering amplitudes. The sign of the magnetic amplitude switches with theH-field direction altering the interference effect. (b) The linear XRIS-H-field dependence is presented by plotting the scattering amplitude at the line indicated energy in (a). The arrows illustrate the spin reorientation of the Eu ions withH-field and the inset shows the measurement (π–π) geometry. The error bars represent the s.d. (c) The energy dependence of the intensity difference between ±0.1 T across the resonance edge with and withoutE-field application (1 × 105V cm−1). The solid line in the top panel is a scaled version of the ±1.2 T data set. The charge–magnetic interference phenomenon is eliminated withE-field. (c—Inset) A microscopic cartoon model of the Eu spin arrangement with and withoutE-field. Naturally, the G-AFM-ordered Eu spins coherently cant towards the externalH-field direction; however, with appliedE-field, the near magnetic degenerate states likely induce a collinear mixed AFM–FM phase devoid of long-range magnetic ordering. While the FM regions produce insufficient coherency themselves, by pining neighbouring AFM spin orientations along the appliedH-field direction they inhibit spin canting and in effect mute the interference effect. S.d. errors are propagated for the difference measurements. Figure 5: The response of Eu spin alignment with applied H -field in the ETO film on LSAT with and without E -field. ( a ) Energy scans through the Eu L II edge at the (003) ETO reflection with ±1.2 T showing the maximum interference effect at full saturation between the magnetic and charge scattering amplitudes. The sign of the magnetic amplitude switches with the H -field direction altering the interference effect. ( b ) The linear XRIS-H-field dependence is presented by plotting the scattering amplitude at the line indicated energy in ( a ). The arrows illustrate the spin reorientation of the Eu ions with H -field and the inset shows the measurement ( π – π ) geometry. The error bars represent the s.d. ( c ) The energy dependence of the intensity difference between ±0.1 T across the resonance edge with and without E -field application (1 × 10 5 V cm −1 ). The solid line in the top panel is a scaled version of the ±1.2 T data set. The charge–magnetic interference phenomenon is eliminated with E -field. (c—Inset) A microscopic cartoon model of the Eu spin arrangement with and without E -field. Naturally, the G-AFM-ordered Eu spins coherently cant towards the external H -field direction; however, with applied E -field, the near magnetic degenerate states likely induce a collinear mixed AFM–FM phase devoid of long-range magnetic ordering. While the FM regions produce insufficient coherency themselves, by pining neighbouring AFM spin orientations along the applied H -field direction they inhibit spin canting and in effect mute the interference effect. S.d. errors are propagated for the difference measurements. Full size image Figure 5c–i presents the XRIS spectroscopic difference applying 0.1 T showing that the magnetic moments cant towards the field direction with ~10% of the full Eu moment. Once the electric field (1 × 10 5 V cm −1 ) is applied, the interference effect is quenched Fig. 5c–ii . This was a surprising result because an enhanced XRIS effect owing to long-range FM order would be expected. Alternatively, if the electric field induced a true AFM–FM degenerate state, such magnetically frustrated moments would nevertheless align along the applied magnetic field direction resulting in an interference effect. Similarly, if the E -field caused a paramagnetic state, 0.1 T is sufficient to align the magnetic moments producing an interference effect owing to small thermal fluctuations at this temperature, 1.9 K. Consequently, the magnetic state induced by the E -field is neither frustrated nor paramagnetic. However, to adequately explain both the XRIS and AFM order suppression would require the emergence of short-range-ordered nanometre-sized FM clustering. This model disrupts the long-range spin coherence of the AFM order while the emergence of FM interactions in short-range cluster formation remains insufficiently large to significantly contribute to the charge–magnetic interference. Our findings present conclusive evidence for direct single-phase cross-field ME control in a compressively strained EuTiO 3 film. Employing in situ X-ray scattering measurements, we present reversible electric switching of magnetic order using a strong intrinsic coupling phenomenon. We have directly measured the microscopic magnetic structure of EuTiO 3 as G-AFM under low-strain states (0.0 and 0.9%) and FM under 1.1% tensile strain. The magnetic critical parameters show −0.9% compressive strain that alters the relative strengths of coexisting AFM and FM magnetic interactions bringing them into competition. First-principles DFT calculations indicate that the third NN Eu ion SE interaction, mediated through the central Ti ion, ultimately determines the G-AFM spin periodicity along the ‹111› direction. Moreover, by calculating the energy of the simulated ETO–LSAT film, we have replicated our experimental findings by modelling the field-induced polarization effect with controlled Ti displacements. As such, the energetic stability of the AFM order dissipates leading to the emergence of FM interactions. The underlying mechanism relies on bond alignment distortion suppressing the efficacy of the third NN Eu–Ti–Eu interaction. This novel ‘giant’ ME coupling phenomenon will likely offer intriguing prospects to explore new types of ME functionality. X-ray resonant magnetic scattering XRMS measurements were performed on the 6-ID-B beamline at the Advanced Photon Source and the XMaS beamline at European Synchrotron Radiation Facility. The sample was mounted on the cold finger of a Joule–Thomson stage closed cycle helium displex refrigerator. The incident X-ray energy at 6-ID was tuned to the Eu L II edge by a liquid nitrogen-cooled double-crystal Si(111) monochromator source with a 3.3-cm period undulator. The XMaS beamline is a bending magnet source, and the energy selection performed with a water-cooled double-crystal Si(111) monochromator. All samples were oriented with respect to the substrate crystallographic axis. The films are epitaxial to their substrates so that the film diffraction peaks are easily found with respect to the substrate reciprocal matrix. The incident X-ray is linearly polarized perpendicular to the scattering plane (σ polarization). The resonant magnetic scattering, arising from electric dipole transitions from the 2 p -to-5 d states, rotates the polarization resulting in π-polarized photons (parallel to the scattering plane). A post-sample pyrolytic graphite analyser at the (0 0 6) PG reflection was used to select π-polarized radiation and suppress the background from charge scattering (σ-polarized light). Magnetic scattering is not frequently used to measure FM with zero magnetic field because the magnetic reflection occurs at the same position in reciprocal space as the larger charge scattered intensity. In the rare-earth compound, however, the magnetic scattering intensity can be comparable to the final charge scattering by coupling the large resonant enhancement and suppression of the charge scattering by polarization analysis [37] . It is expedient to choose the optimum reflection to maximize the magnetic to charge scattering ratio as the chemical structure factor is different from the magnetic structure factor. The (0 0 Odd) ETO charge reflection is about 40 times smaller than the (0 0 Even) ETO reflection, where the diffracted X-rays are in-phase enhancing the scattering amplitude owing to the structure factor of the ETO film. The magnetic structure factor, on the other hand, is the same for both (0 0 Even) ETO and (0 0 Odd) ETO reflections. Hence, we obtained the clear resonant behaviour from the difference between the intensity of the (001) ETO reflection above and below T C presented in Fig. 2b . X-ray resonant interference scattering Measurement of ferromagnetic order can also be achieved from the interference between magnetic and charge scattering at the resonant edge [36] . Nominally in the XRMS process, the electric dipole resonance is dominant. The magnetic scattering (E1 transition) from the moments out of the scattering plane produce the same polarization as the charge scattering when the incoming polarization is parallel to the scattering plane (π polarization). Thus, the charge scattering and magnetic scattering can interfere, and consequently the interference effect is dependent on the magnetic moment direction. X-rays from synchrotron radiation are linearly polarized (in the plane of the synchrotron itself) so by using horizontal scattering geometry with the magnetic field applied in the vertical direction orthogonal to both the beam direction and beam polarization one may measure the interference change by alternating the H -field direction. First-principles DFT We performed DFT calculations with projector-augmented wave potentials in the GGA+U (refs 39 , 40 ) framework, using VASP [41] , [42] code. We used a 8 × 8 × 8 k-point grid for Brillouin zone integrals and a 500 eV plane-wave energy cutoff. This cutoff has been increased to 600 eV in certain parts of the calculations for greater accuracy. Geometric relaxations are done by keeping the in-plane lattice parameter ‘a’ fixed and relaxing the out-of-plane lattice parameter ‘c’. Residual force threshold was decreased to 0.5 eV Å −1 where necessary in order to resolve differences between states close in energy. An external stress has been applied along the c axis in order to compensate for the overestimation of cell volume. Exchange parameters for an Ising model are fitted to total energy calculations done in a 2 × 2 × 2 perovskite supercell that consists of 40 atoms and 10 different magnetic configurations. S.d.’s of these exchange parameters are not reported as they are small and of no qualitative significance. EuTiO 3 is predicted to be near a magnetic phase transition as a function of the on-site Hubbard repulsion parameter U (ref. 30 ). In order to pick a best initial estimate of U , we calculate the Curie–Weiss constant and Neel temperature for bulk (under fixed stress boundary conditions) ETO, the results are presented in Table 2 . It is not possible to reproduce the exact transition temperatures from first principles owing to limitations of the simple mean field theory we used, and also because of the very small energy differences under consideration. However, if we pick a U that gives a T N : T C ratio close to experiment ( T C is extracted from susceptibility measurements [38] ), then we can get a good sense of the competition between FM and AFM states. We see that U =5.7 eV, which is the value that was used in previous studies works well when oxygen rotations were not taken into account [24] . However, once the rotations are taken into account and calculations are repeated in the relevant structure (I4/mcm), a U =5.7 eV overestimates the T N : T C ratio. To better fix the deficiencies in DFT, we instead use U =6.2 eV as standard. Also, an intra-atomic exchange parameter J =1.0 eV is kept fixed. Table 2 T C and T N from first-principles for bulk ETO in space group Pm3m and with varying U for I4/mcm. Full size table How to cite this article: Ryan, P. J. et al . Reversible control of magnetic interactions by electric field in a single-phase material. Nat. Commun. 4:1334 doi: 10.1038/ncomms2329 (2013).